Measured Canadian oil sands CO2emissions are higher than estimates made using internationally recommended methods The oil and gas (O&G) sector represents a large source of greenhouse gas (GHG) emissions globally. However, estimates of O&G emissions rely upon bottom-up approaches, and are rarely evaluated through atmospheric measurements. Here, we use aircraft measurements over the Canadian oil sands (OS) to derive the first top-down, measurement-based determination of the their annual CO 2 emissions and intensities. The results indicate that CO 2 emission intensities for OS facilities are 13–123% larger than those estimated using publically available data. This leads to 64% higher annual GHG emissions from surface mining operations, and 30% higher overall OS GHG emissions (17 Mt) compared to that reported by industry, despite emissions reporting which uses the most up to date and recommended bottom-up approaches. Given the similarity in bottom-up reporting methods across the entire O&G sector, these results suggest that O&G CO 2 emissions inventory data may be more uncertain than previously considered. The objective of limiting the increase in global temperature to <1.5 °C this century is dependent upon reducing anthropogenic greenhouse gas (GHG) emissions to net zero [1] . Identifying mitigation potentials to achieve this goal and assessing GHG reductions relies upon accurate emission estimates of anthropogenic sources, which inform national and international climate policies. Consequently, participating countries in the United Nations Framework Convention on Climate Change (UNFCCC) are required to submit sector-based emissions data in an annual national GHG inventory report (NIR) [2] , [3] . Such anthropogenic GHG emission data ultimately underpin carbon pricing and trading policies. The global energy industry alone accounts for ≈35% of anthropogenic GHG emissions (using a 100-year global warming potential (GWP)) [4] , a significant portion of which are attributed to the global upstream oil and gas (O&G) sector. It is estimated that the global O&G sector (which is included in NIRs) contributes ~10% of anthropogenic GHG emissions [4] , using GHG emission estimates that are derived primarily through complex calculations based upon UNFCCC inventory guidelines [5] . The estimation of anthropogenic GHG emissions in NIRs from stationary sources in the energy sector (including the O&G sector) is primarily a bottom–up exercise, where GHG emissions from individual sources within a given facility are added together, as outlined in UNFCCC protocols [5] . These estimates have varying degrees of accuracy (i.e., Tier 1–3) [5] but fundamentally rely on emission factors and associated activity data (e.g., production and consumption intensity), which in some cases may be outdated or assumed to be homogeneous across the world. In general, Tier 3 approaches are considered to use the best available data specific to the industry and should provide improved emissions estimates relative to Tier 1 and Tier 2 methods. The large contribution of the O&G sector to global GHG emissions underscores the need for accurate sectoral GHG emissions in national inventories. This is particularly relevant since studies have indicated discrepancies between top–down and bottom–up estimates of O&G methane (CH 4 ) [6] , [7] , [8] , [9] , [10] , [11] , [12] , many of which having shown that official inventories or industrial reports underestimate emissions. However, few atmospheric measurement-based evaluations have been performed for O&G carbon dioxide (CO 2 ) emission inventories, despite CO 2 emissions being significantly larger than CH 4 . This may be in part because uncertainties in emission factors and activity data used in bottom–up CO 2 estimates for this sector are considered small (<10%) [5] compared to CH 4 (50–150%) [5] . Nonetheless, small uncertainties in CO 2 emission estimates have the potential to result in large unaccounted for CO 2 based upon the magnitude of the CO 2 emitted compared to CH 4 . Evaluating GHG emissions reported to inventories for the O&G sector is especially important now, with global fossil fuel production and demand at an all-time high [13] . Such evaluations are highly important for countries with resource-based economies such as Canada, where O&G activities account for ≈26% of national GHG emissions and oil sands (OS) production in particular ≈10% [14] . In general, CO 2 emissions from the O&G sector (including the Canadian OS sector) are derived for inventories using an Intergovernmental Panel on Climate Change (IPCC) Tier 3 approach [15] and following the UNFCCC protocols [16] . However, estimates of the emission intensity (kg CO 2 e per barrel of oil) of OS operations and of their absolute GHG emissions are not derived from direct measurements of CO 2 . Aircraft measurements over large-scale O&G emission sources can provide a top–down assessment of these bottom–up reported GHG estimates. Here the utility of a top–down measurement approach is demonstrated below for the Canadian OS surface mining operations (one of the largest single O&G sources of GHGs in Canada). The results indicate that overall, OS GHG emissions may be underestimated and suggests that reporting that follows this Tier 3 approach (or less accurate Tier 1 and Tier 2 approaches) may universally underestimate CO 2 emissions. This highlights the potential need for updated IPCC inventory guidelines that include atmospheric measurement-based evaluations of CO 2 emissions, for an improved assessment of the O&G contribution to the global anthropogenic GHG burden. 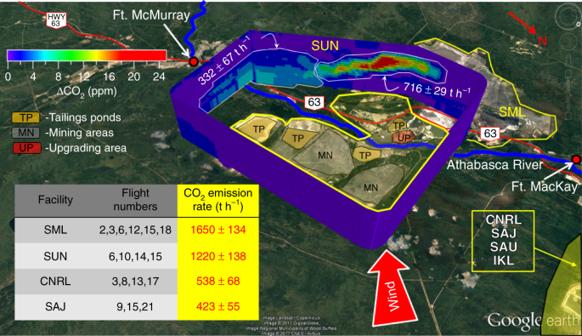Fig. 1 Measured CO2from flight 15 around the SUN facility. Mass emission rates have been determined for this facility using the TERRA algorithm, where elevated and surface emissions can be quantified separately. The mean hourly CO2emission rates (t h−1) during all flights covering the four major surface mining operations in the oil sands are shown in the inset table. Uncertainties represent the standard error\(\left( {\frac{\sigma }{{\sqrt N }}} \right)\)for the multiple flights over a facility. Map data: Google, Image Landsat, CNES/Airbus, Digital Globe 2017. Source data for the inset table are provided in Supplementary Data1 Hourly emission rates Thirteen aircraft flights around the OS surface mining facilities in Alberta (Supplementary Table 1 ) were conducted in the summer of 2013, with virtual polygon flight boxes surrounding a given facility that encompassed all CO 2 emission sources, including mining, processing, upgrading, and tailings release [17] (Supplementary Fig. 1a–c ). Approximately 5–12 different altitudes were flown for each box, depending upon the facility. Background subtracted CO 2 data from these flights were used as inputs into a Top–down Emissions Rate Retrieval Algorithm (TERRA) [18] (see Methods), from which hourly CO 2 emission rates were derived. For the OS surface mining facilities, an example virtual box is shown in Fig. 1 for the Suncor (SUN) facility and the resultant hourly CO 2 emissions for all facilities in the inset table. The downwind side of the virtual box of Fig. 1 demonstrates the complexity of CO 2 plumes from this facility including emissions from both ground sources and elevated stacks, which can be quantified separately. Based on these flights, the largest hourly CO 2 emissions are associated with Syncrude Mildred Lake (SML; 1650 ± 134 t h −1 ) and SUN (1220 ± 138 t h −1 ) facilities, followed by Canadian National Resources Ltd Horizon (CNRL; 538 ± 68 t h −1 ) and Shell Albian and Jackpine (SAJ, now part of CNRL, 423 ± 55 t h −1 ), all of which are dominant compared to CO 2 from local transportation within the virtual box (see Supplementary Note 1 ). Propagated uncertainties (see Methods) associated with hourly emission rates for single flights were small (≈8–26%; Supplementary Table 1 ), with emission rates consistent between flights (relative standard error (RSE) ≈ 8–13%; Fig. 1 ) despite being conducted on various days spanning approximately 1 month. Fig. 1 Measured CO 2 from flight 15 around the SUN facility. Mass emission rates have been determined for this facility using the TERRA algorithm, where elevated and surface emissions can be quantified separately. The mean hourly CO 2 emission rates (t h −1 ) during all flights covering the four major surface mining operations in the oil sands are shown in the inset table. Uncertainties represent the standard error \(\left( {\frac{\sigma }{{\sqrt N }}} \right)\) for the multiple flights over a facility. Map data: Google, Image Landsat, CNES/Airbus, Digital Globe 2017. Source data for the inset table are provided in Supplementary Data 1 Full size image Emission intensities For each surface mining facility, the CO 2 emission intensity \(( {I_{{\mathrm{CO}}_2}} )\) , in units of \({\mathrm{kg}}_{{\mathrm{CO}}_2}{\mathrm{barrel}}^{ - 1}\) of synthetic crude oil (SCO), is shown in Fig. 2a . The \(I_{{\mathrm{CO}}_2}\) is derived by upscaling the hourly CO 2 emissions (Fig. 1 , Supplementary Table 1 ) to monthly values (see Methods) and dividing by known monthly facility production volumes of SCO [19] . The overall lifecycle GHG emission intensity for any petroleum source is dominated by the combustion of its end product (e.g., gasoline), which is relatively constant and accounts for 70–80% of the total GHG emission [20] . Hence, to compare the GHG emission across various petroleum sources, estimates typically only include processes occurring from the well to the refinery gate (WTRG) and are based on quantities derived from various emission models [21] , [22] , [23] . The current results are the first top–down WTRG estimates of \(I_{{\mathrm{CO}}_{2}}\) for the OS using direct CO 2 measurements, thus providing a benchmark for the assessment of previous model estimates of \(I_{{\mathrm{CO}}_{2{\mathrm{eq}}}}\) (which include CH 4 ). Such model estimates are known to be highly variable, due mainly to the types of sources included in the model, uncertainties in fuel-related assumptions, and other methodological challenges [20] , [24] , [25] , [26] . The derived \(I_{{\mathrm{CO}}_2}\) here ranged from 44.3 ± 6.8 to 245 ± 25.4 \({\mathrm{kg}}_{{\mathrm{CO}}_2}{\mathrm{barrel}}^{ - 1}\) (Fig. 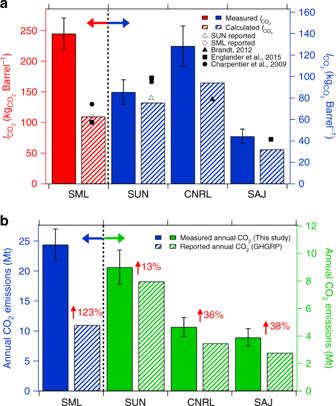Fig. 2 CO2emission intensities and total emissions.aAircraft measurement derived (mean) and calculated well to the refinery gate CO2emission intensities\((I_{{\mathrm{CO}}_2})\)for the 4 major surface mining operations in the oil sands in 2013 (n=3–6). Calculated emission intensities use publically available data from the GHG reporting program (GHGRP) for the same facilities (2013). Opaque data points represent facility-specific model calculation of\(I_{{\mathrm{CO}}_{2{\mathrm{eq}}}}\)in the literature and open symbols represent\(I_{{\mathrm{CO}}_{2{\mathrm{eq}}}}\)reported directly by the industry for 2013. SAJ (now part of CNRL) does not upgrade to synthetic crude oil on site, hence its intensity is per barrel of bitumen. The\(I_{{\mathrm{CO}}_2}\)for SML includes emissions from SAU.bAnnual emissions of CO2measured for the four major surface mining facilities in 2013 compared to those reported by industry to the GHGRP. Error bars ina,brepresent the propagated uncertainty of the mean value. Source data are provided in Supplementary Data1 2a and Supplementary Table 2 ) for the 4 major surface mining facilities in operation in 2013. Including measurement-based CH 4 emissions reported previously [12] in the present CO 2 emissions results in \(I_{{\mathrm{CO}}_{2{\mathrm{eq}}}}\) ranging from 47.6 ± 7.6 to 267 ± 31 \({\mathrm{kg}}_{{\mathrm{CO}}_{2{\mathrm{eq}}}}{\mathrm{barrel}}^{ - 1}\) , which is dominated by the contribution from CO 2 (see Methods). With the exception of SML (which includes emissions of SAU), the measured \(I_{{\mathrm{CO}}_{2{\mathrm{eq}}}}\) are somewhat larger than the \(I_{{\mathrm{CO}}_{2{\mathrm{eq}}}}\) calculated using overall industry average inputs from up to 6 years earlier (77–122 \({\mathrm{kg}}_{{\mathrm{CO}}_2}{\mathrm{barrel}}^{ - 1}\) SCO) [25] . However, the measured \(I_{{\mathrm{CO}}_{2{\mathrm{eq}}}}\) here does not include the emissions associated with transport of SCO to the refinery gate. Including such emissions would make the actual \(I_{{\mathrm{CO}}_{2{\mathrm{eq}}}}\) even larger than industry average model values [20] , [25] , [26] . The difference between estimated and reported intensities is even larger when comparing the currently estimated \(I_{{\mathrm{CO}}_2}\) (or \(I_{{\mathrm{CO}}_{2{\mathrm{eq}}}}\) ) with those reported for specific facilities in the same year (2013). In this case, the estimated \(I_{{\mathrm{CO}}_2}\) are 13–123% larger than those calculated using CO 2 emissions reported to Environment and Climate Change Canada’s GHG reporting program (GHGRP) [15] and reported production volumes [19] (see Methods). The measurement-based \(I_{{\mathrm{CO}}_2}\) values are similarly larger than the \(I_{{\mathrm{CO}}_{2{\mathrm{eq}}}}\) provided directly by industry [27] , [28] for 2013 (Fig. 2a ). The estimated \(I_{{\mathrm{CO}}_2}\) for SUN is in reasonable agreement with the calculated estimates shown in Fig. 2a , being only 13% higher and within the measurement uncertainty. In contrast, estimates of the mean \(I_{{\mathrm{CO}}_2}\) for CNRL, SAJ, and SML/SAU are 36%, 38%, and 123% greater than those calculated using publicly available data [15] , [19] and larger than the facility-specific \(I_{{\mathrm{CO}}_{2{\mathrm{eq}}}}\) modeled in recent studies [24] , [25] , [26] . Fig. 2 CO 2 emission intensities and total emissions. a Aircraft measurement derived (mean) and calculated well to the refinery gate CO 2 emission intensities \((I_{{\mathrm{CO}}_2})\) for the 4 major surface mining operations in the oil sands in 2013 ( n = 3–6). Calculated emission intensities use publically available data from the GHG reporting program (GHGRP) for the same facilities (2013). Opaque data points represent facility-specific model calculation of \(I_{{\mathrm{CO}}_{2{\mathrm{eq}}}}\) in the literature and open symbols represent \(I_{{\mathrm{CO}}_{2{\mathrm{eq}}}}\) reported directly by the industry for 2013. SAJ (now part of CNRL) does not upgrade to synthetic crude oil on site, hence its intensity is per barrel of bitumen. The \(I_{{\mathrm{CO}}_2}\) for SML includes emissions from SAU. b Annual emissions of CO 2 measured for the four major surface mining facilities in 2013 compared to those reported by industry to the GHGRP. Error bars in a , b represent the propagated uncertainty of the mean value. Source data are provided in Supplementary Data 1 Full size image Annual emission estimates Based upon the aircraft-estimated \(I_{{\mathrm{CO}}_2}\) , the annual CO 2 emissions for each facility are estimated (see Methods) and shown in Fig. 2b , together with the CO 2 emissions reported by industry to the GHGRP for 2013. The aircraft measurement-based annual CO 2 emissions from the 4 major OS facilities ranged from 3.9 ± 0.6 to 25 ± 3 Mt. 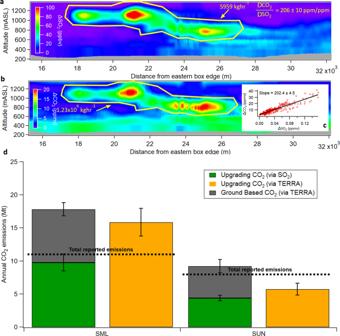Fig. 3 Emissions of CO2for upgrading operations and ground-based sources in the oil sands.aBackground subtracted SO2in elevated plumes from OS upgrading emissions during flight 18 derived with TERRA.bBackground subtracted CO2in the same elevated plumes of flight 18.cDirect correlation between background subtracted CO2and SO2within plumes.dAnnual emissions of CO2from upgrading stacks for SML and SUN derived using the CO2:SO2emission ratios measured in plume (green bars; see Methods). Orange and gray bars represent upgrading and ground-based emissions, respectively, derived using TERRA directly and up-scaled as described in Methods. Dashed lines represent total facility-reported CO2emissions to the GHG reporting program. Error bars in Fig.2a, brepresent the propagated uncertainty of the mean value. Source data are provided in Supplementary Data1 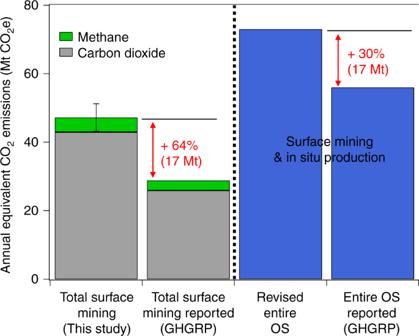Fig. 4 Total oil sands (OS) annual greenhouse gas (GHG) emissions compared to those reported to the GHG reporting program. Methane emissions from Baray et al.12are added to the surface mining CO2measured here, to be comparable to reported\({\mathrm{CO}}_2{\mathrm{e}}\). A global warming potential (GWP) of 25 is used for methane. Blue bars include in-surface and in situ OS extraction. Revised estimate for total OS emissions includes the measured surface mining emissions determined in this study and the reported emissions from in situ operations. Errors associated with annual CO2(Fig.2b) and CH4estimates have been added in quadrature:\(\delta = \sqrt {\delta _{{\mathrm{CO}}_2}^2 + \delta _{{\mathrm{CH}}_4}^2}.\)Source data are provided in Supplementary Data1 These emissions are higher than the reported CO 2 emissions, reflecting the differences in the aircraft measurement-estimated vs facility-estimated \(I_{{\mathrm{CO}}_2}\) , with the largest statistically significant difference (see Methods) of 13 Mt year −1 for SML/SAU (123%) and the smallest for SUN (13%). The differences between aircraft-estimated and facility-reported CO 2 emissions for SML and SUN are further validated through a separate approach using measurements of sulfur dioxide (SO 2 ) and reported mined OS ore volumes [19] as tracers for stack and ground-based CO 2 emissions, respectively (see Methods). For these two facilities, the emissions of SO 2 are associated with bitumen upgrading and are generally confined to elevated stack outflows only, leading to elevated SO 2 plumes downwind (Fig. 3a , Supplementary Fig. 2 ). Hence, CO 2 plumes from both these facilities are clearly split into an elevated stack plume that is closely associated with the SO 2 plume and a ground-based plume (Fig. 3b ). Multiplying the CO 2 to SO 2 emission ratios in the elevated plumes (Fig. 3a, c ) with measured annual SO 2 emissions [29] provides an alternative means to determine annual stack CO 2 emissions specifically (Fig. 3d ) (See Methods and Supplementary Note 2 ). Similarly, a ground-based emission ratio was estimated by normalizing the TERRA-derived ground-based emissions by the monthly volume of mined OS ore (see Methods). Using these approaches, the separated annual CO 2 emissions from stacks and ground emissions at SML are estimated at 14.2 ± 1.3 and 8.1 ± 1.0 Mt, respectively (Fig. 3d ). This result is consistent with that derived using TERRA specifically for elevated plumes (Fig. 3d ) and indicates that stack CO 2 emissions alone are ~29% greater than the reported facility total CO 2 emissions for SML/SAU (all sources; Fig. 3d ). Furthermore, the combined emissions (stacks + ground based; 22.3 ± 3.5 Mt) for SML are in agreement with the facility total derived above through the use of \(I_{{\mathrm{CO}}_2}\) (24.5 ± 3.0 Mt, which includes SAU; Fig. 2b ), supporting the discrepancy between total aircraft measurement-based estimated and total reported CO 2 emissions for this facility (Fig. 2b ). In contrast, stack CO 2 emissions estimated for SUN are ~20% lower than the reported facility total CO 2 emissions (all sources; Fig. 3d ), while the total measured stack (6.4 ± 0.4 Mt)+ground CO 2 emissions (4.8 ± 0.7 Mt) are only slightly higher than the reported CO 2 emissions of Fig. 2b . Based on Fig. 3d , it is estimated that stack CO 2 emissions for SML and SUN account for 61 ± 12% and 67 ± 13% of their respective total emissions, in relative agreement with available model estimates [20] , [24] . Fig. 3 Emissions of CO 2 for upgrading operations and ground-based sources in the oil sands. a Background subtracted SO 2 in elevated plumes from OS upgrading emissions during flight 18 derived with TERRA. b Background subtracted CO 2 in the same elevated plumes of flight 18. c Direct correlation between background subtracted CO 2 and SO 2 within plumes. d Annual emissions of CO 2 from upgrading stacks for SML and SUN derived using the CO 2 :SO 2 emission ratios measured in plume (green bars; see Methods). Orange and gray bars represent upgrading and ground-based emissions, respectively, derived using TERRA directly and up-scaled as described in Methods. Dashed lines represent total facility-reported CO 2 emissions to the GHG reporting program. Error bars in Fig. 2a, b represent the propagated uncertainty of the mean value. Source data are provided in Supplementary Data 1 Full size image The overall impact of the differences between measured and reported GHG emissions found here is large. Put into context, the unaccounted emissions represent a total CO 2 e (100-year GWP timescale) emission increase of ~64% (or 17 Mt year −1 ) over that reported for OS surface mining operations (Fig. 4 ) and a ~30% increase for the entire OS (including reported in situ emissions) (Fig. 4 ). Such an absolute emission quantity (17 Mt year −1 CO 2 e) is similar to the GHG emissions from a metropolitan area the size of Seattle [30] or Toronto [31] . Additionally, GHG emission reports from OS in situ extraction facilities have yet to be evaluated using atmospheric measurements. This suggests that the potential exists for further unaccounted GHG emissions, as partially demonstrated by Lagrangian flights that show hourly CO 2 emissions downwind that are larger than the sum of individual facility emission rates (see Supplementary Note 3 ). Fig. 4 Total oil sands (OS) annual greenhouse gas (GHG) emissions compared to those reported to the GHG reporting program. Methane emissions from Baray et al. [12] are added to the surface mining CO 2 measured here, to be comparable to reported \({\mathrm{CO}}_2{\mathrm{e}}\) . A global warming potential (GWP) of 25 is used for methane. Blue bars include in-surface and in situ OS extraction. Revised estimate for total OS emissions includes the measured surface mining emissions determined in this study and the reported emissions from in situ operations. Errors associated with annual CO 2 (Fig. 2b ) and CH 4 estimates have been added in quadrature: \(\delta = \sqrt {\delta _{{\mathrm{CO}}_2}^2 + \delta _{{\mathrm{CH}}_4}^2}.\) Source data are provided in Supplementary Data 1 Full size image There are important implications associated with the current findings. Since many stationary combustion sources in the O&G sector derive their emissions using similar Tier 1–3 protocols [5] , this issue may not be unique to the OS or to CO 2 . Indeed, the Tier 3 approach (and other provincial reporting regulations) used for the OS is considered to utilize the best possible data, and yet top–down and bottom–up results here remain significantly different. This may suggest that other GHG sources or industries in other regions, which use less accurate bottom–up methods (i.e., Tier 1) could exhibit similar discrepancies between top–down and bottom–up estimates. The results here further suggest that top–down emission estimates can be used to inform the development of federal and provincial emission regulations and highlights the value of atmospheric measurements in tracking and/or monitoring progress in terms of emission reduction targets. Equally important is that the underlying data used in reporting to the GHGRP are also used in formulating OS GHG emission estimates in Canada’s NIR to the UNFCCC [16] . Both the GHG emission estimates in the GHGRP and NIR are considered Tier 3 according to the IPCC as they use the best available information specific to the industry and provide the highest possible accuracy [5] , [16] . As a result, the GHGRP and NIR emission data vary little from each other for specific facilities, with uncertainties associated with OS fugitive CO 2 emissions [16] , overall emissions for the Canadian energy sector [16] , and stationary combustion emission factors [5] reported as approximately ±6%, ±3%, and ±< 10%, respectively. However, the top–down measurement results here indicate that the total inventory GHG estimates for the OS sector may need to be revised upward by at least 30%. Most importantly, the results imply that complex emission factors and activity data used in NIRs should be periodically re-assessed and highlights the potential need for new IPCC guidelines for atmospheric measurement-based validation of emissions. Such guidelines are particularly important since atmospheric measurements are now recognized for their ability to systematically monitor GHG emissions in support of the Paris Agreement [32] . Finally, this type of atmospheric observation can directly inform stakeholders at the subnational scale about unknown or poorly quantified GHG sources at the facility level, as a contribution to the recently adopted integrated global GHG Information System [33] of the World Meteorological Organization and United Nations Environment Program. Aircraft measurements Aircraft measurements of CO 2 and CH 4 over the Athabasca OS region of northern Alberta were performed from August 13 to September 7, 2013 as part of an intensive field campaign. Details of the study objectives, aircraft implementation, and other technical aspects have been described previously [17] , [34] . During the study, 22 flights totaling 84 h were conducted over individual facilities of the OS and downwind of the facilities at distances up to 120 km. The flight patterns have been shown previously [17] , 13 of which were used to quantify primary emissions from individual OS facilities, and 4 conducted to quantify their transformation downwind. Emission quantification flights were conducted by flying a 4- or 5-sided polygon, at multiple altitudes, resulting in 21 separate virtual boxes encompassing 7 OS facilities. Results from 17 flights were used in the current analysis, while the others were excluded because of highly variable wind speeds and direction and/or the presence of confounding pollutant interferences from adjacent OS facilities. The specific facilities studied and their corresponding flight numbers are given in Supplementary Table 1 . Three of the flights (F7, F19, and F20) examined the photo-chemical transformation of pollutants downwind of the OS facilities [34] and are used here to quantify total emissions from all OS surface mining facilities (for comparison to the sum of individual emission flights), as they encompass the majority of emissions from the region. These transformation flights were designed as Lagrangian, such that the same air parcel in the OS plumes was sampled successively, 1 h apart, in virtual screens constructed from level flight tracks at multiple altitudes (Supplementary Fig. 3 , Supplementary Table 1 ). There were no industrial emissions between the screens of each flight. Gas, particle, meteorological, and aircraft state measurements were made during flights, with a detailed description provided elsewhere [17] , [34] , [35] . The current work makes use of a subset of these measurements specifically for the quantitation of CO 2 and SO 2 gases. CO 2 was measured using a Picarro model G2401- m instrument ( http://www.picarro.com/products_solutions/gas_analyzers/flight_co_co2_ch4_h2o ) with a time resolution of 2 s [12] . The instrument sampled ambient air through a 6.35-mm (1/4 inch) diameter perfluoroalkoxy, backwards facing sampling line with a residence time of ~2 s. Calibrations were performed before, during, and after the field campaign using a range of mixing ratios from NIST certified standard cylinders (350–450 ppm). The precision of the CO 2 measurements in flight were estimated to be <100 ppb. SO 2 was measured using a Thermo Scientific 43iTLE analyzer with a time resolution of 1 s. The SO 2 instrument was calibrated with NIST certified standard cylinders over a range of 0–400 ppb. The standard deviation of the calibration slopes was 0.9% and the average standard deviation of the 1-s data during calibrations was 1.99 ppb [18] . The time delay for the SO 2 measurement, due to the gas traversing the length of the inlet, was ≈6 s and was corrected for in the data. NO and NO 2 measurements were made using two Thermo Scientific 42iTLE analyzers at 1 Hz (NO X averaged to 2 s) with a sample residence time of ≈3–4 s. Each instrument was calibrated with NIST standard cylinders of NO. High frequency wind data were averaged to 1 or 2 s for subsequent analysis in the emission rate algorithm. Top–down emission rate retrieval algorithm analysis CO 2 emission rates for each OS surface mining facility and for the entire OS region were derived using an algorithm designed to estimate pollutant transfer rates through the virtual boxes/screens of aircraft measurements. The algorithm is based on the Divergence Theorem to resolve mass balance (TERRA) [18] and has been used extensively for determining emission rates of volatile organic compounds (VOCs), black carbon, CH 4 , secondary organic aerosol (SOA), organic/inorganic acids, and SO 2 [17] , [18] , [34] , [36] Emissions are derived with the TERRA algorithm by combining box-like aircraft flight patterns with pollutant concentration measurements at high time resolution and wind speed and direction data. The algorithm applies simple kriging [18] to the data to produce virtual walls of gridded 20 × 40 m 2 mesh on the virtual box, resolves the air mass balance within the virtual box, and determines the mass transfer rates across the walls (including the top of the box) to derive a net emission rate for a pollutant. In the case of virtual screens (rather than boxes), TERRA quantifies the mass transfer rate of a pollutant (kg h −1 ) through the virtual screens, in the same manner as it does for a single wall of a virtual box flight [34] , [36] . The use of the standard TERRA to estimate emissions accounts for incoming and outgoing air mass advective and turbulent fluxes within a volume, including the top of the virtual box, and is ideal for species that have little background contribution to the measured concentration. However, in the case of CO 2 that has a large background concentration, this approach can introduce large uncertainties if even a small portion of the measured CO 2 is calculated to leave through the top of the box. To address this uncertainty, a background CO 2 is subtracted prior to the use of TERRA, such that the transfer rate through any one outgoing side of a box (or single screen) represents the facility emission rate. This approach has been used successfully for CH 4 [12] , VOCs [35] , [36] , and SOAs [34] and is similar to other single screen approaches [37] , [38] . Background CO 2 was determined using upwind measurements for box flights and screen flights (where available). For screen flights where upwind measurements were not conducted, the levels at the edges of the screen were used as background. The background between upwind data was linearly interpolated and box-car smoothed within a 20–40-min moving window to derive a variable baseline CO 2 for the entire 2–3 h flight. Examples of the derived CO 2 baseline are shown in Supplementary Fig. 3 . The uncertainty added to the final emission rate for each flight contributed by the baseline estimation method was examined by varying the derived CO 2 baseline by the standard deviation of the upwind data (±0.5–3 ppm CO 2 ), followed by input into TERRA. This baseline CO 2 sensitivity analysis resulted in CO 2 emission rates that varied by 1–33% ( δ B ; Supplementary Table 1 ). This relatively small variation in emission rates caused by the background CO 2 is due to the short duration of the flights, which were flown during an established planetary boundary layer and because there was significant enhancement of plume CO 2 of up to >80 ppm above background. In general, a changing boundary layer depth could in principle introduce additional uncertainty in the emission results from TERRA. However, the flights were intentionally conducted during mid-afternoon hours, when the boundary layer was constant. This was assessed through vertical profiles performed before and after the emission estimation portions of the flights. Under conditions where boundary layer depth was stable, real-time vertical profile data (pollutants, water vapor, temperature) from the flights were used to ensure that the highest flight track was always above the top of the boundary layer, hence ensuring that the entire plume from the various facilities was contained within the specific flight box or within the flight screen. It has been demonstrated previously that extrapolation of pollutant concentrations from the lowest flight level to the ground is the main source of uncertainty in TERRA, with an overall uncertainty in the derived emission rates of approximately 20% [18] . This was determined previously [18] through a sensitivity analysis in a series of closed-loop numerical experiments. In such experiments, a simulated Gaussian plume driven by a known emission flux was created and sampled with the TERRA algorithm, while also using various forms of extrapolation to the ground (i.e., linear to the ground, exponential, constant, linear to zero). A similar analysis was performed in the current study, with the differences in extrapolations also resulting in a <20% difference in final estimated emissions. For pollutant sources that are entirely above the lowest flight level, extrapolation to the ground is not relevant and the associated uncertainty in the TERRA-derived emissions has been demonstrated to be ≈ 4% [18] . This was determined by comparing the TERRA-derived emissions of SO 2 with continuous emissions monitoring system (CEMS) data for the same facility stack (CNRL) and for the exact hour of the flight. We note that CEMS data are regularly audited and mandated to be accurate to within 10%. Further comparisons of TERRA-derived SO 2 stack emission rates with those concurrently measured with CEMS indicate that this uncertainty may be even smaller (<1%) as shown in Supplementary Fig. 4a . However, the larger 4% uncertainty for elevated stack emissions is used in this analysis. The excellent agreement between TERRA emissions and the audited CEMS data provide confidence that uncertainties associated with possible under sampling are negligible. The uncertainties for stack and ground-based emissions (i.e., 4% and 20%) are applied separately in cases where low level and elevated stack sources are clearly spatially differentiated, which are further propagated with the uncertainties associated with the background CO 2 determination described above. The overall propagated uncertainty associated with the hourly emission rates derived for individual facilities ranged from 8% to 28% \((\Delta E_{{\mathrm{CO}}_2})\) for facility flights and from 24% to 38% for downwind transformation flights as shown in Supplementary Table 1 . In contrast to the emission box flights, the largest uncertainty in the transfer rates through the downwind screens arises from the background subtraction of CO 2 ( δ B in Eq. 9 below) due to the higher variability in background CO 2 over a typically longer flight time. Such uncertainties are included in the emission results from TERRA and reported separately in Supplementary Table 1 . Upscaling OS emissions The hourly emissions of CO 2 derived with TERRA in Fig. 1 and Supplementary Table 1 are used to calculate the CO 2 emission intensity \(\left( {I_{{\mathrm{CO}}_2}} \right)\) for individual facilities ( \({\mathrm{kg}}_{{\mathrm{CO}}_2}{\mathrm{barrel}}^{ - 1}\) SCO) as a first step to estimating annual CO 2 emissions. This emission intensity is derived as 
    I_CO_2 = E_M_CO_2/P_SCO
 (1) where \(E_{{\mathrm{M}}_{{\mathrm{CO}}_2}}\) is the measured emission rate of CO 2 for a given facility scaled to a month and P SCO is the reported monthly production volume of SCO in units of barrels (reported to the Alberta Energy Regulator (AER)). Since production volumes are reported as monthly totals [19] , the measured hourly emission rates ( \(E_{{\mathrm{CO}}_2}\) ) must be scaled up to a month to be used in the above equation (see below). The fact that the relative standard deviation between flights for a single facility spanning a period of a month was <10% supports this monthly upscaling of emission rates. Alternatively, production volumes and hourly CO 2 emissions can both be scaled to daily values. For simplicity, we have chosen to only scale the emissions measurements to monthly values; however, scaling both the emissions up and the production down to 1 day results in the same CO 2 intensities (within <1%). Scaling the hourly CO 2 emissions to daily or monthly values with a simple 24 h (i.e., 1 day) or 744 h (i.e., 1 month) scaling factor may overestimate the total emissions during that time period. Rather, we have used an approach described previously for VOC emissions [17] . As described in Li et al., the TERRA-derived hourly emission rates are converted to daily (or monthly) emission rates based on the diurnal (or monthly) changes in bitumen production. This approach is ideally suited to CO 2 as it is not likely to have the added complexity of temporally/temperature-dependent emissions from non-combustion sources, which may not scale with production. For combustion-based emissions, the hourly emission rate ( E m ) is related to the average hourly emission rate ( \(\overline {E_{\mathrm{m}}}\) ), the hourly bitumen production q at the hour of measurement, and the 24-h production p . E_m = 24 ∗E_m( q/p)
 (2) Since combustion and thus production is accompanied by NO X emissions, the ratio q / p may be derived as 
    ( q/p) = E_NO_X/∑ E_NO_X
 (3) where \(E_{{\mathrm{NO}}_X}\) is the hourly emission rate during aircraft measurement, and \(\mathop {\sum }\nolimits E_{{\mathrm{NO}}_X}\) is the daily NO X emission rate. Thus a factor C daily , for converting hourly to daily emission rates, can be expressed as 
    C_daily = 24 ∗q/p = 24 ∗ E_NO_X/∑ E_NO_X
 (4) Similarly, a scaling factor to convert hourly to monthly emission rates is derived as 
    C_monthly = 744 ∗ E_NO_X/∑ E_NO_X
 (5) where \({\sum} {E_{{\mathrm{NO}}_X}}\) is the monthly emission rate. Using NO X as an indicator of production is convenient since hourly, daily, and monthly NO X emission rates are available from CEMS measurements. The underlying assumption is that both CO 2 and NO X emissions are proportional to SCO production, which is consistent with the fundamental assumptions for emission factor-based emission reporting, and consistent with the empirical relationship between CO 2 and NO X observed here (Supplementary Fig. 4b ). Although various in-plant sources of combustion exist, each with a different NO X /CO 2 ratio, this assumption requires the aggregate NO X emissions (sum of all CEMS data) to vary with production. While SO 2 was chosen previously as a surrogate for production [17] , we have chosen to use NO X , as the CEMS data for NO X is more likely to include other stack combustion sources in addition to the upgrader stacks, which are the main source of SO 2 . While it is not known whether the NO X /CO 2 ratios from different sources within a facility are temporally invariant, the standard deviation of the slope of the empirical relationships in Supplementary Fig. 4b are used as a measure of the potential error introduced by variable NO X /CO 2 ratios during the study ( δ V ). The CEMS data for \(E_{{\mathrm{NO}}_X}\) from the facilities are reported to be accurate to within 10% [39] ( δ CEM ). The uncertainty in each C monthly scaling factor per flight ( δ C ) is then derived as 
    δ _C = √(2(δ _CEM^2) + δ _V^2)
 (6) and ranged from ≈14% to 15%. The mean scaling factor C monthly is derived to be 0.83 ± 0.05, 1.00 ± 0.07, and 0.89 ± 0.06 for SML, SUN, and CNRL, respectively. For other facilities where no CEMS data were available, the average of the terms above is used to calculate C monthly (0.91 ± 0.13). The monthly CO 2 emission rates ( \(E_{{\mathrm{M}}_{{\mathrm{CO}}_2}}\) ) for a given facility are then derived as 
    E_M_CO_2 = E_CO_2×744/C_monthly
 (7) where \(E_{{\mathrm{CO}}_2}\) is the TERRA-derived hourly emission rate (720/ C monthly is used for September) . This is subsequently used to compute the CO 2 emission intensities \(( {I_{{\mathrm{CO}}_2}} )\) via Eq. ( 1 ) above and shown in Fig. 2a and Supplementary Table 2 . Annual OS CO 2 estimates and uncertainties Annual CO 2 emissions ( E annual ) for individual facilities are derived by multiplying the top–down derived CO 2 emission intensities (Supplementary Table 2 ), by the reported annual SCO production volumes for the year 2013 [19] : 
    E_annual = I_CO_2× P_SCO_annual
 (8) The derived annual CO 2 emissions have an overall relative error ( δ E ) with contributions from the errors associated with the application of TERRA ( δ T ≈ 7–20%), the baseline CO 2 estimation ( δ B ≈ 1–20%), the hourly to monthly scaling factor ( δ C ≈ 14–15%; above), the relative measured variability in TERRA-derived emissions from multiple flights per facility (standard error; δ D ≈ 4–10%), and the reported production volumes of SCO ( δ P ≈ 1%). The overall relative uncertainty in the annual emission rate ( δ E = ΔE annual / E annual ) can hence be calculated as 
    δ _E = √(δ _T^2 + δ _B^2 + δ _C^2 + δ _D^2 + δ _P^2)
 (9) for each flight and ranged from 17% to 32% depending on the facility (Supplementary Table 2 ). The mean annual emissions (across individual flights) for each facility is shown in Fig. 2b , with the error bars representing the propagated uncertainty of the mean (see Supplementary Table 2 ). The uncertainty associated with the calculated emission intensities \(( {I_{{\mathrm{CO}}_2}} )\) of Fig. 2a are also derived with Eq. ( 9 ), but using a value of δ P (≈ 1%) for monthly reported production (rather than annual production). This also results in a calculated uncertainty in \(I_{{\mathrm{CO}}_2}\) of 17–32%. The absolute uncertainties in \(I_{{\mathrm{CO}}_2}\) derived for each individual facility flight are provided in Supplementary Table 2 and ranged from ±10 to ±76 kg CO 2 barrel −1 , with a propagated error in the mean \(I_{{\mathrm{CO}}_2}\) for each facility ranging from ±7 to ±26 kg CO 2 barrel −1 (see Supplementary Table 2 ). It is expected that applying the emission intensities \(( {I_{{\mathrm{CO}}_2}} )\) derived for 1 month in this study across the entire year to determine annual emissions is significantly more accurate than attempting to scale the measured CO 2 emissions from these flights directly to a full year. This intrinsically assumes that the measured emission rates are more representative of a month than they are to a full year and only requires \(( {I_{{\mathrm{CO}}_2}} )\) to be relatively constant from month to month (see other considerations and assumptions section). Annual CH 4 emissions used in Fig. 4 were taken directly from previous work [12] . Deriving an emission intensity for methane (to be included in the total \(I_{{\mathrm{CO}}_{2{\mathrm{eq}}}}\) ) using similar upscaling factors as was done for CO 2 may not be fully appropriate for CH 4 , as most CH 4 in the OS is not derived via combustion. Hence \(I_{{\mathrm{CO}}_{2{\mathrm{eq}}}}\) for CH 4 specifically was derived by dividing previously reported annual CH 4 [12] by annual production volumes of SCO [19] . Regardless, applying the upscaling approach for CO 2 described above to hourly CH 4 resulted in CH 4 emission intensities that differed by <5% and remain a small contributor to overall OS GHG emissions (using 100-year GWP). The statistical significance of the differences between reported annual CO 2 emissions and those derived here (Fig. 2b ) are investigated through the use of a single-sample t test, since as with all reported emissions there is only a single reported value for each facility. This analysis tests the null hypothesis that can be stated as: \(\bar M\) = μ o , i.e., the mean of all aircraft measurement results for a given facility ( \(\bar M\) ) equals the reported value ( μ o ). Consequently, the t statistic can be given as: 
    t = M̅ - μ _o/√(∑X^2 - ( ( ( ∑X)^2)/N)/( N - 1)N)
 (10) where \(\bar M\) is the sample mean, μ o is the reported value, X are the aircraft-based emission rates from all flights of a facility, and N is the number of flights for each facility, with a degree of freedom of N − 1. Using this test for the SML facility results in a t = 8.4, which translates into a p value of 0.0004. This indicates that the aircraft measurement-based emission results for SML are statistically and significantly different from the reported emission at the 99.9% confidence level. The results for other facilities resulted in t values of 1.95, 2.32, and 2.69 for SUN, CNRL, and SAJ, respectively. This corresponds to means that are different than reported values at p < 0.2, <0.1 and <0.1 (i.e., ~80–90% confidence level). Other considerations and assumptions There are potentially additional considerations that should be noted with respect to the estimated emission intensities and annual emissions particularly when compared to traditional bottom–up approaches. Such bottom–up approaches rely upon accurate and detailed knowledge of: the technology in use, emission factors, fuel mixture data, operating conditions, quality of maintenance, control technologies in use, carbon content data, and the lower or higher heating values (LHV vs HHV) of the process. These items can have a degree of uncertainty associated with them and do not include the potential for unintentional errors or omissions of sources (among the very many bottom–up sources that exist). While aircraft measurements of CO 2 concentrations and associated top–down methodologies are also subject to a range of quantifiable uncertainties, the approach provides a useful and complimentary dataset to bottom–up methods, which can identify when further investigation into emissions is required, particularly when discrepancies exist. While it is not possible to unequivocally determine the root causes of the observed discrepancies here, it is speculated that that they may arise from a combination of factors, including outdated emission factors and activity data, unknown/poorly updated fuel carbon content data, poorly quantified area sources, and human error. Such difficulties are expected to be faced by various O&G and other industries, suggesting the potential for universal differences between top–down and bottom–up emission estimation methods. Some additional uncertainties for the top–down methodology (those not already stated in methods) are also possible. For example, the aircraft measurements were performed over the course of a month and appropriately scaled, taking into account monthly production to derive emission intensity. A seasonal change in emission intensity during non-sampled months is possible, although we expect that this should be minimal (<15%) as noted previously [26] , particularly since seasonal emissions of CO 2 from fugitive sources such as tailing ponds are small contributors to overall CO 2 emissions [40] . Since much of the CO 2 is a result of combustion, it expected that increased energy/heat would be required during the winter, potentially resulting in increased emission intensities compared to the summer. In addition, changes in the fuel mixture used within facilities over the year can influence the derived emission intensities. For example, increased use of pet coke as fuel (which is known to emit more CO 2 ) during the month of this study could bias the derived emission intensities high compared to other months. The underlying assumption in this regard is that the relative proportion of fuel types used during the aircraft flights was similar to other months. This is supported by OS plant statistics [19] , which show that the fraction of pet coke used varied by <10% month to month in 2013 for SML. Regardless, the carbon content of pet coke is only 10–15% higher than that of natural gas and process gas used for fuel and would only apply to 60–70% of total facility emissions (i.e., not from the mining process). Other end products arising from OS operation (i.e., not SCO) are also possible, which could introduce some uncertainty into the emission intensity estimates that use SCO production in the denominator of the equation for \(I_{{\mathrm{CO}}_2}\) . This is also expected to be relatively small as SML and SUN generally produce ~90% SCO [26] . Regardless, using an alternative emission factor approach (i.e., CO 2 /SO 2 or CO 2 /ore mined) results in very similar annual emissions compared to the emission intensity approach. The results from these independent approaches are good evidence that they are valid and support the underlying assumption that NO X emissions on aggregate are proportional to SCO production (see Methods). Regardless, provided that the product mixture does not change significantly from month to month, the derived \(I_{{\mathrm{CO}}_2}\) remains a valid emission factor that can be used to calculate annual emissions. The OS plant statistics [19] support the assumption of a constant product mixture as it varies by <10% month to month. Finally, the possibility of unforeseen facility maintenance, open burning of overburden, or increased flaring resulting in increased CO 2 emissions cannot be ruled out. However, there was no evidence of maintenance or burning occurring during this study, and flaring is expected to account for a very small fraction of the overall CO 2 emissions. Regardless, such events are unlikely to have occurred systematically across the exact days of study during the months of August and September. Reporting summary Further information on experimental design is available in the Nature Research Reporting Summary linked to this article.